Site-selective hexa-hetero-functionalization of α-cyclodextrin an archetypicalC6-symmetric concave cycle Access to C n ( n >4) symmetric cyclic concave molecules with a different function on each of their n subunits is an unmet challenge. The reason lies in the lack of a post-functionalization method whose site selectivity is sufficiently understood, predictable and modulable to access most functionalization patterns. Here we disclose a new site-directing rule for a debenzylation reaction on cyclodextrins that solves this problem and allows the unprecedented access to penta- and ultimately hexa-differentiations of such C 6 concave cycles. This achievement opens the access to objects with very high-density information. The repartition of atoms in space through chemical bonding is the essence of synthetic chemistry. Chemists developed this ability over time allowing the conversion of small molecules into larger and ever more complex molecular architectures. The understanding and mastering of the rules of what could be once called a handcraft allowed its conversion into an art, the ‘art of total synthesis’ with so impressive achievements that they can be pointed out as master-pieces [1] . This field induced the discovery of many new chemical transformations, the development of enantioselective synthesis being a striking example. Another approach consists in derivatizing pre-existing molecules in the diversity of structures offered by Nature. This approach also called semisynthesis has its own impressive realizations, the best illustration being certainly the famous story of taxol. This anti-cancer molecule is found in very low quantities in the bark of yews, so low, that its extraction could threaten the survival of the species. Its semisynthesis from an intermediate, 10-deacetyl baccatin III, abundantly found in the leafs of the same trees allowed its industrial production [2] . The key in this transformation is the selective reaction of each of the four free hydroxyl groups of 10-deacetyl baccatin III exploiting their innate reactivity differences. Central to this field is the ability to discriminate between functions and/or regions of the molecule, i.e., to achieve chemoselective and/or regioselective reactions, respectively. In other words, site-selectivity is the great challenge. This frontier area ultimately aims to transform any group on a given molecule based on their innate reactivity [3] and the tuning of the reagent properties. Some steps towards this goal have been taken in particular with the regioselective C–H activations on complex molecules [4] , [5] , [6] , but also the selective functionalization of reactive functions such as OH groups [7] , [8] , [9] , or the regioselectivity in cyclization reactions [10] , [11] . Site-selective reactions occur because small differences in chemical environment, that is, electronic and/or steric properties pre-exist. But there are molecules, which are strictly symmetrical, for which it is thus necessary to create those differences. This is the case of an important family of compounds: the cyclic concave molecules, which are at the root of supramolecular host-guest chemistry but also find applications in daily life and industry. These include naturally occurring cyclodextrins (CDs), but also synthetic compounds such as calixarenes, cucurbituryls, resorcinarenes, pillararenes, bambusurils, asararenes and so on. Those molecules built upon n identical subunits possess a C n symmetry that hampers their selective functionalization because of the absence of innate reactivity difference between subunits. Furthermore, most of the time the individual units are isolated electronically from one another; therefore, the difference in reactivity has to rely solely on sterics and more generally on arrangement in space of the reactive sites. In fact, the very high majority of functionalizations of such molecules consists in the addition of one new function once [12] , [13] , [14] , [15] , [16] , [17] , [18] , [19] or on all equivalent reactive sites. Even the addition of the same function twice has been the subject of intense research in the past 30 years or so [20] , [21] . The extreme difficulty of the poly-hetero-functionalization of C n symmetric molecules lies in the figures given by combinatorics: for a cycle of C 6 symmetry with six functionalizable sites there are 14 ways to arrange two functions, 130 ways to arrange three functions, 700 ways to arrange four functions, 2,635 ways to arrange five functions and 7,826 ways to arrange six functions. The arrangements of n beads of k colours can be generated on http://www.jasondavies.com/necklaces/ , which corresponds to the well-known combinatorics problem of necklaces [22] . In practice, that means that reacting a C 6 functionalizable molecule with six different reagents of equal reactivity statistically leads to a mixture of 7,826 differently functionalized molecules, ranging from 6 molecules bearing six times the same substituent to 120 molecules with six different substituents. 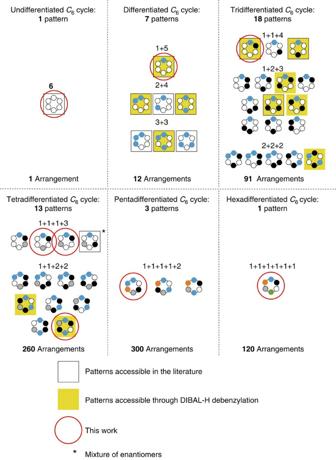Figure 1: Functionalization patterns. Schematic representation of all the possible functionalization patterns forC6concave cycles, each unit of the molecule is represented as a dot, if two units of the molecule bear two different functions, the dots have different colours. Below each collection of patterns the number of arrangements of the corresponding number of functions is indicated, for example, there are 300 arrangements of exactly five colours on six positions (seeSupplementary Discussion). Figure 1 shows the patterns of colour arrangements on a C 6 cycle that are classified according to the number of colours and translated in terms of differentiation of various reactive positions on a molecule. For sake of clarity, only the patterns are displayed and not all the arrangements. As an example, in the differentiated (2 different colours) section, we drew one blue ball plus five white ones, but not the one with five blue balls and one white, which is equivalent in terms of patterns, but which constitutes a totally different species if one thinks of a molecule with two different functions. Thus, the number of possible arrangements is given below each section. The patterns of functionalization that have already been reported in the literature for all kinds of C 6 symmetric concave cycles are also indicated. It clearly appears that most differentiated cycles are now available. This relatively simple problem of regioselectivity, namely getting a single product out of 14, which could otherwise be separated [23] , has been the prime challenge in this area for the past few decades. In the field of CDs, seminal work by Tabushi and Knowles paved the way to compounds with two [24] or three [25] identical functions in the 1970s and developed in the next 30 years [20] , [21] , but heterofunctionalization of CDs was only accomplished after difficult separation of mixtures of regioisomers [26] , [27] . It is only recently that strategies to get concave molecules with more than two different functions emerged. For instance a tridifferentiated C 4 resorcinarene, with three different groups, was synthesized en route to superbowl containers [28] . Tridifferentiated calix(4)arenes were also synthesized as racemic mixtures because of their inherent asymmetry [29] , [30] , [31] . In the realm of molecules of higher symmetry, C 6 calix(6)arenes with three [32] , [33] or even four [34] functionalities (tetradifferentiated) have also been described albeit inherently as racemic mixtures. Regarding CDs, tridifferentiated compounds are accessible mainly through three methods: regioselective opening [35] , [36] , [37] or formation [38] of bridged-CDs, imidazolyl-directed sulfonation [39] and regioselective debenzylation [40] , [41] , [42] . Tetradifferentiation has also been achieved using the last two methods [39] , [43] , [44] . Figure 1: Functionalization patterns. Schematic representation of all the possible functionalization patterns for C 6 concave cycles, each unit of the molecule is represented as a dot, if two units of the molecule bear two different functions, the dots have different colours. Below each collection of patterns the number of arrangements of the corresponding number of functions is indicated, for example, there are 300 arrangements of exactly five colours on six positions (see Supplementary Discussion ). Full size image This quick survey clearly shows a void in the literature: a method whose site directing effects are sufficiently understood, predictable and modulable to access most functionalization patterns, the ultimate challenge being the access to a hexadifferentiated C 6 concave cycle, a task out of sight with current available methodologies. Here we disclose a new site-directing rule for the debenzylation reaction on CDs that allows the unprecedented construction of penta- and hexadifferentiated concave cycles. This achievement opens avenues to objects with very high-density information. Site-directing rules To meet this challenge, it is necessary to delineate enough predictable directing effects for the functionalization of CDs. For some time now we have been developing methods to hetero-functionalize CDs based on the understanding of the mechanism of a deprotection reaction. This reaction is a debenzylation reaction discovered serendipitously [45] , [46] and operated by diisobutylaluminium hydride (DIBAL-H) leading to CD A,D-diol 3 from perbenzylated CD 1 (ref. 47 ). The mechanism of the reaction involves the chelation of the aluminium reagent between the primary and the endocyclic oxygen atoms of a glucopyranosidic unit as shown in CD 4 ( Fig. 2 ). Furthermore, the double deprotection is a stepwise process, because it is possible to isolate monol CD 2 and react it to produce A,D-diol 3 again. Therefore, the first deprotection site-directs the second through steric hindrance of the aluminoxyde on intermediate 5 ( Fig. 2 ). 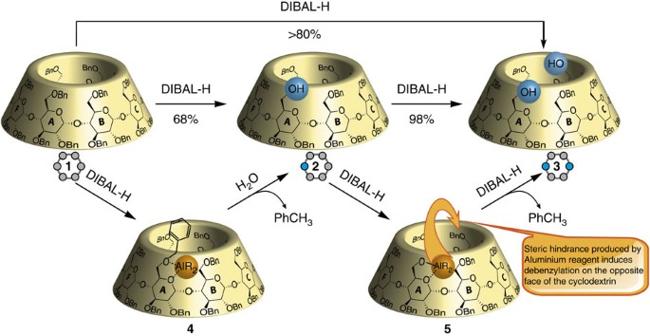Figure 2: Basic regioselective DIBAL-H deprotection of benzylated cyclodextrins. Per-benzylated CD1affords monol CD2or diol CD3depending on the reaction conditions. Under the action of DIBAL-H, monol CD2is converted into diol CD3, indicating that the first deprotection orients the second one through steric hindrance induced by the aluminium reagent as shown on CD5. Approach of DIBAL-H on sugar A is hampered by the presence of benzyloxy on position 6 of sugar B as shown on CD4. Figure 2: Basic regioselective DIBAL-H deprotection of benzylated cyclodextrins. Per-benzylated CD 1 affords monol CD 2 or diol CD 3 depending on the reaction conditions. Under the action of DIBAL-H, monol CD 2 is converted into diol CD 3 , indicating that the first deprotection orients the second one through steric hindrance induced by the aluminium reagent as shown on CD 5 . Approach of DIBAL-H on sugar A is hampered by the presence of benzyloxy on position 6 of sugar B as shown on CD 4 . Full size image This breakthrough allowed us to devise an easy and selective access to tridifferentiated CDs, and only recently did we report a route to tetradifferentiated ones. Hence, we have developed two different ways to site-direct a second debenzylation of functionalized CDs built on the reaction mechanism. In a first instance, we have shown that an azido group on sugar A of benzylated CD 6 was directing a debenzylation reaction mediated by DIBAL-H on the diametrically opposed sugar D to give CD 7 (ref. 40; Fig. 3a ) This directing effect was attributed to the crowding induced by the attachment of the aluminium reagent to the nitrogen during the primary azide reduction in a similar way as in the conversion of 2 in 3 . In a second instance, we showed that steric decompression on the primary rim of the CD, caused by a vinyl group on sugar A of CD 8 , directed the deprotection reaction on the adjacent clockwise (viewed from the primary rim) sugar F to give CD 9 . This directing effect is the consequence of both the cyclic directionality of the CD, and the asymmetric effect of the substituents of neighbouring sugars on the approach of the aluminium reagent. This can be seen on CD 4 where the aluminium atom on unit A lies in the region of the benzyloxy group of the counterclockwise (view from top) sugar B ( Fig. 2 ). Reversely, suppressing the benzyloxy group in sugar A as in 8 favoured approach of Al on its clockwise unit F to give 9 . This decompression could be accomplished in two ways either through replacement of the benzyloxy group in sugar A by less crowded methyl or vinyl groups as in 8 giving the clockwise F-monol 9 ( Fig. 3b ) or by bridging two diametrically opposed glucose units A and D as in CD 10 to give C,F-diol 11 (ref. 41; Fig. 3c ). A higher degree of complexity was reached through combination of both methods, in a ‘frustration’ strategy, where a 6-vinyl sugar D was placed opposite to azido-derived sugar A in CD 12 , the action of DIBAL-H afforded an unexpected tetradifferentiated CD C,E-diol 13 (ref. 44; Fig. 3d ). This combination of rules allowed the access to tetradifferentiated CDs in a very regioselective manner. However, this route is a dead-end towards hexadifferentiation of CDs, on the way of which we need to pass through a CD exhibiting three new functions added once each. The monofunctionalization of diol 13 would only lead to a statistical mixture of products. In fact, five site-directed mono-debenzylations are necessary to access the ultimate hexadifferentiated functionalization pattern. 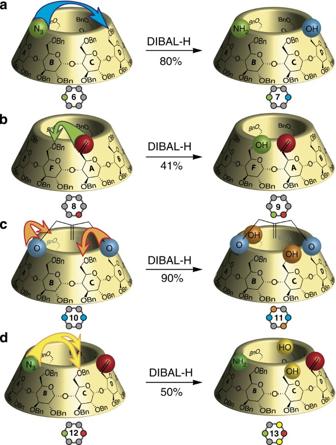Figure 3: Site-directing debenzylation effects on CDs. (a) A-azido CD6undergoes a tandem azide-reduction/O-debenzylation on the diametrically opposed sugar D to give CD7. (b) A vinyl group on sugar A of CD8induces a clockwise deprotection on sugar F to give CD9. (c) A,D-bridged CD10undergoes a double clockwise deprotection to afford C,F-diol CD11. (d) A frustrated A-azido, D-vinyl CD12undergoes a double deprotection on both sides of the vinyl group to give C,E-diol CD13. Figure 3: Site-directing debenzylation effects on CDs. ( a ) A-azido CD 6 undergoes a tandem azide-reduction/ O -debenzylation on the diametrically opposed sugar D to give CD 7 . ( b ) A vinyl group on sugar A of CD 8 induces a clockwise deprotection on sugar F to give CD 9 . ( c ) A,D-bridged CD 10 undergoes a double clockwise deprotection to afford C,F-diol CD 11 . ( d ) A frustrated A-azido, D-vinyl CD 12 undergoes a double deprotection on both sides of the vinyl group to give C,E-diol CD 13 . Full size image Dissymmetrical bridge as a new site-directing tool To reach that goal, we reasoned that we could combine our two rules in a different manner. Bridging A-amino,D-alcohol CD 7 could produce a dissymmetrical bridge with a sterically decompressed ether side D and a functionalizable secondary amine side A. Functionalization of the amine side A with a bulky group would prevent deprotection in its vicinity on sugar F and induce the desired third mono-deprotection only on sugar C. Hence, A-amino,D-alcohol CD 7 was methallyl-bridged to afford CD 14 in 55% yield. The amine in sugar A was further derivatized with a benzyl group to give 15 in 96% yield. Much to our disappointment, subsequent treatment with DIBAL-H only yielded either a mixture of compounds or a C,F-diol 17 (65% yield) upon prolonged reaction time corresponding to a bis clockwise debenzylation. Use of a bulkier protecting group such as 3,5-di-tert-butylbenzyl did not induce any preferred deprotection affording C,F-diol 18 in 73% yield from CD 16 . Paradoxically, a regioselective mono-deprotection on sugar C was observed starting from unprotected A-amino,D-ether bridged CD 14 yielding CD 19 in 62% yield. The corresponding C,F-diol 20 could be obtained only under more forcing conditions ( T >60 °C, N 2 flux, longer reaction time), albeit in a rather moderate 42% yield ( Fig. 4 ). 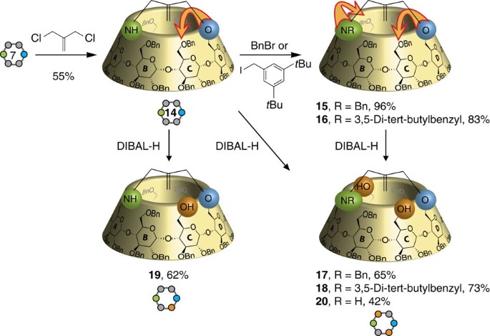Figure 4: Site-directing effect of an amino-ether bridge. A-amino,D-hydroxy CD7is methallyl bridged to give CD14. If the amine is protected as in CDs15and16DIBAL-H induces a double clockwise C,F-deprotection to give CDs17and18, respectively. If the amine of the bridge is not further protected as in CD14, DIBAL-H only induces a monodeprotection on sugar C clockwise to the ether moiety of the bridge on sugar D to give CD19. Complete experimental details and characterization are supplied inSupplementary Methods. Figure 4: Site-directing effect of an amino-ether bridge. A-amino,D-hydroxy CD 7 is methallyl bridged to give CD 14 . If the amine is protected as in CDs 15 and 16 DIBAL-H induces a double clockwise C,F-deprotection to give CDs 17 and 18 , respectively. If the amine of the bridge is not further protected as in CD 14 , DIBAL-H only induces a monodeprotection on sugar C clockwise to the ether moiety of the bridge on sugar D to give CD 19 . Complete experimental details and characterization are supplied in Supplementary Methods . Full size image At first glance, this result violates the established directing rules mentioned above: the debenzylation occurs next to a bulky tertiary amine and not next to the secondary amine. We therefore hypothesized that DIBAL-H was complexing the secondary amine congesting the region surrounding the amine. The clockwise deprotection is then eased at the ether terminus of the bridge rather than next to the aluminium adduct. To sustain this proposal, we reacted the secondary A-amine 21 with DIBAL-H, and observed a clean formation of the expected diametrically opposed A-amino,D-hydroxy CD 22 in 65% yield. This regioselectivity derives from the directing effect of a first DIBAL-H molecule interacting with the secondary amine on sugar A producing 23 , and inducing the usual steric orientation of the second DIBAL-H on the diametrically opposed sugar unit D. ( Fig. 5 ) The difference in bulk between a diisobutyl aluminium adduct and a benzyl group indeed accounts for the difference in reactivity between CDs 14 and 15 . 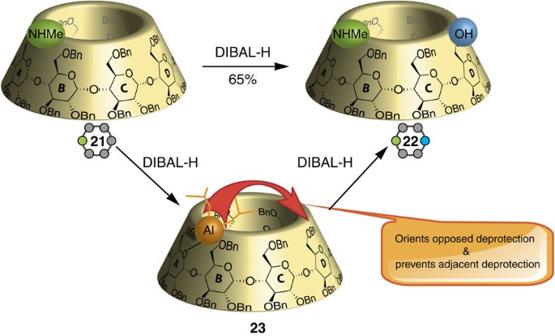Figure 5: Secondary amine site-directing effect through attachment of an aluminium reagent. When secondary amine-CD21is reacted with DIBAL-H, a diametrical deprotection occurs on ring opposite sugar D to give22. This indicates that the aluminium reagent attaches to the amine to give23to operate a site-direction through steric hindrance. Figure 5: Secondary amine site-directing effect through attachment of an aluminium reagent. When secondary amine-CD 21 is reacted with DIBAL-H, a diametrical deprotection occurs on ring opposite sugar D to give 22 . This indicates that the aluminium reagent attaches to the amine to give 23 to operate a site-direction through steric hindrance. Full size image Synthesis of hexadifferentiated CDs This breakthrough allowed us to plan the synthesis of the ultimately hexadifferentiated CD, displaying one unique functional group on each sugar unit. The first monodebenzylation was operated on perbenzylated CD 1 , to give monodifferentiated CD 2 in 64% yield [43] . The free alcohol on sugar A was oxidized to the corresponding aldehyde and olefinated to afford the A-vinyl CD 8 in 90% yield. According to our previously established rules, sterically decompressed CD 8 underwent regioselective DIBAL-H-mediated debenzylation on sugar unit F adjacent to sugar A bearing the vinyl group to give CD 9 in 41% yield (64% based on recovering starting material) [43] . The hydroxyl group in tridifferentiated CD 9 was converted into an azido group using conventional procedures. The F-azido, A-vinyl CD 24 underwent a tandem azide-reduction/ O -debenzylation reaction to afford the expected tetradifferentiated F-amino, C-hydroxy, A-vinyl CD 25 in 78% yield. Methallyl bridging of CD 25 gave the C,F-capped CD 26 (72%), which was monodebenzylated to give pentadifferentiated CD 27 in 56% yield, deprotection occurring on adjacent sugar B and clockwise to the ether moiety of the bridge following the new site-directing rule. The next step consisted in the duplication of the tandem reaction, that required amine protection in sugar F to avoid association with aluminium, which prevents efficient adjacent deprotections, as shown in the case of CD 14 ( Fig. 4 ). In contrast, F-amino, B-azido CD 28 exclusively gave the diametrically opposed B-amino, E-hydroxy CD 29 in 70% yield, the first hexadifferentiated CD bearing six different functional groups on its primary rim that is one different function on position 6 of each sugar units ( Fig. 6 ). 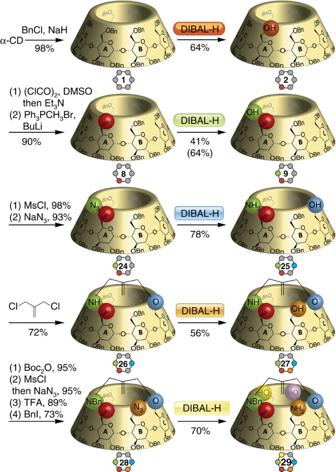Figure 6: Hexadifferentiation of α-CD through five successive site-directed DIBAL-H mono-debenzylations. Complete experimental details and characterization are supplied inSupplementary Methods. Figure 6: Hexadifferentiation of α-CD through five successive site-directed DIBAL-H mono-debenzylations. Complete experimental details and characterization are supplied in Supplementary Methods . Full size image Further chemical transformation of hexadifferentiated CD 29 allows the synthesis of CD 30 possessing six orthogonal functions: amine, alkene, azide, alcohol, ether and chloride. The reactions sequence consisted in the Boc-protection of the amine, chlorine substitution of the alcohol, deprotection of the bridge and azidation of the amine ( Fig. 7 ). It is also possible to form another regioisomeric hexadifferentiated CD 32 using a different order of reactions starting from pentadifferentiated CD 28 . Hence, bridge-deprotection, azidation of the formed primary amine, methylation of the secondary amine and conversion of the hydroxyl group into a chloride affords pentadifferentiated CD 31 starting from CD 28 . CD 31 possesses five orthogonally functionalizable sites. Finally, action of DIBAL-H to operate a tandem azide reduction and diametrically opposed debenzylation affords hexadifferentiated CD 32 regioisomeric to CD 30 after azidation ( Fig. 7 ). 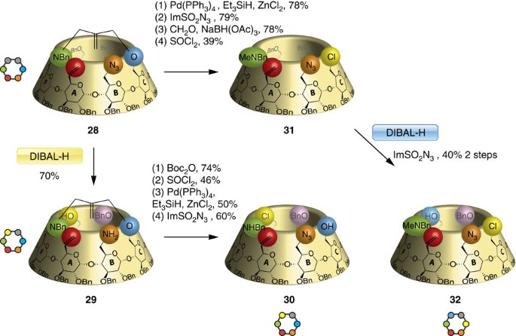Figure 7: Protecting group manipulation of penta- and hexadifferentiated α-CDs. Complete experimental details and characterization are supplied inSupplementary Methods. Figure 7: Protecting group manipulation of penta- and hexadifferentiated α-CDs. Complete experimental details and characterization are supplied in Supplementary Methods . Full size image We now have in hand an ensemble of rules for the site-directed debenzylation of polybenzylated CDs that demonstrated its versatility in the accomplishment of the ultimate hexadifferentiation of this class of C 6 concave cycles. Incidentally, we also synthesized a pentadifferentiated CD, a level of complexity unreached before, and accessed two new tetradifferentiation patterns. We thus believe that our method is able to accomplish on-demand polyheterofunctionalization of CDs. Considering that monofunctionalization itself tremendously expanded the range of applications of CDs, it is easily foreseeable that increasing the degree of functionalization on molecules able to include guests and self-assemble will lead to objects with high-density information, which may find applications in areas as diverse as theragnostics, energy and smart materials. Synthesis Synthesis of all compounds are described in detail in Supplementary methods . Structure determination All new compounds were thoroughly characterized by NMR spectroscopy, rigorously establishing the pattern of functionalization, see Supplementary Figs 1–26 , Supplementary Tables 1–6 and Supplementary Methods . As a characteristic example, the detailed NMR analysis of hexadifferentiated CD 29 is given in the Supplementary Discussion . How to cite this article: Wang, B. et al. Site-selective hexa-hetero-functionalization of α-cyclodextrin an archetypical C 6 -symmetric concave cycle. Nat. Commun. 5:5354 doi: 10.1038/ncomms6354 (2014).